Clinical relevance of molecular characteristics in Burkitt lymphoma differs according to age While survival has improved for Burkitt lymphoma patients, potential differences in outcome between pediatric and adult patients remain unclear. In both age groups, survival remains poor at relapse. Therefore, we conducted a comparative study in a large pediatric cohort, including 191 cases and 97 samples from adults. While TP53 and CCND3 mutation frequencies are not age related, samples from pediatric patients showed a higher frequency of mutations in ID3 , DDX3X, ARID1A and SMARCA4 , while several genes such as BCL2 and YY1AP1 are almost exclusively mutated in adult patients. An unbiased analysis reveals a transition of the mutational profile between 25 and 40 years of age. Survival analysis in the pediatric cohort confirms that TP53 mutations are significantly associated with higher incidence of relapse (25 ± 4% versus 6 ± 2%, p-value 0.0002). This identifies a promising molecular marker for relapse incidence in pediatric BL which will be used in future clinical trials. Burkitt lymphoma (BL) and its leukemic manifestation Burkitt leukemia (B-AL) is the most common subtype of non-Hodgkin lymphoma (NHL) in children and adolescents accounting for ~50% of cases. In comparison, BL only accounts for 1% of adult NHL cases in Europe and Northern America [1] , [2] , [3] , [4] . The genetic hallmark of BL is a translocation involving the MYC oncogene and the immunoglobulin loci, primarily immunoglobulin heavy chain (IGH) in 80% of cases [t(8;14)(q24;q32)]. Variant MYC translocations involve the light chain loci [t(8;22) or t(2;8)] [5] . Aside from MYC translocations, somatic single-nucleotide variants, insertions, and deletions (SNV/indels) of the ID3-TCF3-CCND3 pathway represent the most frequent genetic events in BL, with up to 90% in pediatric cases, but significantly lower frequency in adult BL [6] , [7] . Recent reports have advanced the molecular understanding of BL biology by identifying additional genetic mutations, revealing genomic and transcriptomic alterations contributing to MYC dysregulation, and tracing the clonal evolution of BL [8] , [9] , [10] , [11] , [12] . But data on the effect of patient age on the molecular characteristics of BL are very limited and show inconclusive results [7] , [13] . With current risk-adapted chemoimmunotherapy, the event-free survival exceeds 90 or even 95% for pediatric cohorts [14] . In contrast, 80% of adult BL patients are cured with multi-agent chemotherapy, and survival rates for younger adults are better [15] , [16] , [17] , [18] . Disease relapse usually occurs shortly after the end of therapy and is associated with a dismal prognosis and survival rates below 30% [14] , [19] , [20] , [21] . Given the poor outcome for patients who relapse, there is a critical medical need for treatment optimization. To this end, targeted approaches and risk-based adaptation of treatment intensity is required. To enable such progress in patient care, translational results based on molecular markers and clinical data are urgently needed. Here, we provide a thorough analysis of the mutational profile of 191 pediatric BL/B-AL by sequencing 134 predefined genes in all samples and by investigating somatic copy number aberrations (SCNAs) in a sub-group of 72 samples. Clinical data were sourced for all 191 cases. These results were compared to the mutational landscape of 97 adult BL cases as there is only limited information about the differences of both age groups [22] . Our analyses identified prognostically relevant genetic lesions of TP53 and GPC5/MIR17HG in pediatric instances, and pinpointed promising targets for BL treatment development in future studies. Clinical characteristics and cohort overview We evaluated 288 patients with confirmed diagnoses of BL or Burkitt leukemia (B-AL or Burkitt lymphoma with a blast count of 25% or more in the bone marrow). In particular, cases with 11q aberration have been excluded, as they are considered a different entity [23] . For the 191 pediatric cases, the median age at diagnosis was 9 years. 30% of pediatric patients were female. Approximately 10% were diagnosed with stage I/II disease, according to the St. Jude staging system, while about 40% had stage III and 50% stage IV disease. 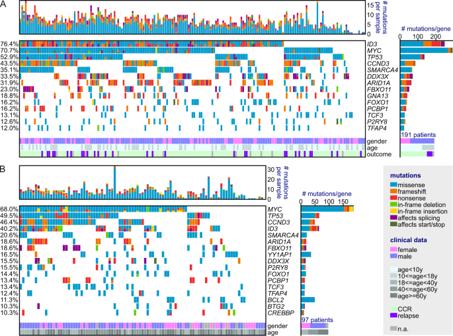Fig. 1: Mutational landscape of pediatric and adult BL. In total, 191 pediatric and 97 adult patient samples were analyzed. Mutations with ≥10% cohort frequency are displayed.AIn total, 14 recurrently mutated genes were found in the pediatric cohort, withID3being the most frequently altered gene. The color code indicates mutation types or clinical data classes (see legend).BIn the adult cohort, 17 recurrently mutated genes were detected. In particular,YY1AP1andBCL2were unmutated or less frequently mutated in the pediatric cohort. The clinical characteristics of the pediatric cohort are summarized in Supplementary Table 1 . The adult cohort comprised 97 cases, with a median age of 52 years at diagnosis, and was 40% female. (Supplementary Data 1 ). 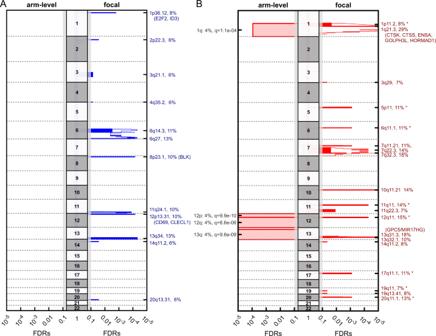Fig. 2: Somatic copy number aberrations (SCNAs). Significant recurring SCNAs are displayed as blocks, based on 72 pediatric cases (55 BL and 17 B-AL cases). Curves indicate residualq-values by GISTIC 2.0 after explaining broad aberrations (Supplementary Data7).AFocal deletions affectingE2F2andID3were detected.BThe most consistently observed SCNA containsGPC5(q= 1.8e-9). Notably, the non-protein-codingMIR17HGcluster directly precedes this gene and is also affected by these gains and amplifications (Supplementary Data6). *: might represent benign (germline) copy number variants. For sample source information, see Supplementary Table 2 . Mutational landscape of pediatric BL We performed targeted next-generation sequencing for fresh-frozen samples, including 86 matched normal tissue for the 191 pediatric cases. To maximize sensitivity and specificity, our analysis pipeline for variant discovery and filtering makes use of several methods and external databases (see Supplementary Fig. 1 and “Methods”). Overall, we identified 1399 SNV/indels for the 191 pediatric cases and 824 SNV/indels in the adult cohort (Supplementary Data 2 ), representing 7.3 and 8.5 alterations per sample, and ranging from 0 to 23 total SNV/indels per case (Supplementary Data 3 ). To test the sensitivity of our pipeline, we additionally performed validation experiments. Only two variants detected by Sanger sequencing in validation regions were not discovered by targeted DNA sequencing, in both cases due to deletions that are likely too long for DNA sequencing to recognize (see validation by Sanger sequencing in “Methods” and validation overview in Supplementary Data 4 ). As another control of our analysis pipeline, we used ten cell lines to verify the concise calling of all SNV/indels (Supplementary Fig 2 ). In the full cohort (pediatric and adult cases combined), the highest frequency of SNV/indels was detected in the MYC gene, with 479 SNV/indels, resulting in 1.7 SNV/indels per case on average, followed by ID3 with 1.1 (Supplementary Data 2 ). Interestingly, MYC showed a higher mutation rate in adults when compared to children, at 1.9 and 1.5 per case, respectively (Supplementary Fig. 3 ). Most of the recurrently mutated genes are involved in regulatory processes and are functionally linked to transcription factor binding ( DDX3X , ID3 , SMARCA4 , TCF3 , and TP53 , Supplementary Table 2 ) or activation of transcriptional processes ( ARID1A , SMARCA4 , TCF3 , TFAP4 , FOXO1, and TP53) . Furthermore, DDX3X , FOXO1 , ID3 , TFAP4, and TP53 are also involved in the regulation of apoptotic processes. Focusing on genes recurrently mutated in at least 10% of cases, 14 were identified in the pediatric cohort (Fig. 1A ) and 17 in the adult cohort. To test whether these genes were positively selected by mutation processes, we applied dNdScv [24] . All genes except one showed a dN/dS ratio significantly higher than one, indicating excess coding mutations (Supplementary Data 5 ). TCF3 was likely not verified only due to alternative transcripts (see “Methods”); mutations were called by strongest consequence logic for TCF3 protein variant 2 (NP_001129611). Interestingly, these recurrently altered genes were significantly different between the two age groups, with YY1AP1 , BCL2 , BTG2, and CREBBP recurrently altered in adult but not pediatric BL cases, while alterations in GNA13 were more predominant to the pediatric cohort (Fig. 1B ). In the pediatric cohort, eight genes ( ID3 , MYC , TP53 , CCND3 , SMARCA4 , DDX3X , ARID1A , and FBXO11 ) were altered in more than 20% of all patient samples, while in the adult cohort only five genes ( MYC , TP53 , CCND3 , ID3 , and SMARCA4 ) were mutated in 20% of cases or more. Fig. 1: Mutational landscape of pediatric and adult BL. In total, 191 pediatric and 97 adult patient samples were analyzed. Mutations with ≥10% cohort frequency are displayed. A In total, 14 recurrently mutated genes were found in the pediatric cohort, with ID3 being the most frequently altered gene. The color code indicates mutation types or clinical data classes (see legend). B In the adult cohort, 17 recurrently mutated genes were detected. In particular, YY1AP1 and BCL2 were unmutated or less frequently mutated in the pediatric cohort. Full size image Recurrent somatic copy number alterations in pediatric BL Using single-nucleotide polymorphism arrays, we analyzed 72 pediatric BL cases for SCNAs via GISTIC 2.0 (Fig. 2 and Supplementary Data 6 ). In all, 4% of all samples were identified as polyploid according to the ASCAT analysis (Supplementary Data 7 ). Chromosomes 1q (4%), 12p (4%), 12q (4%), and 13q (4%) were mostly affected by arm level amplifications. Remarkably, deletions were detected less frequently in our analysis. For a specific region that only contains the protein-coding gene GPC5 (chr13:91398619-92867237), we identified recurrent gains (8.4%) or amplification (9.5%) in 18% of patients (Fig. 2 ). Investigating this locus in detail revealed that the directly preceding miR17-92 cluster is also affected by these copy gains or amplifications ( MIR17HG at chr13:91347820-91354575, which was shown before ; cluster comprised of MIR17 , MIR18A , MIR19A , MIR20A , MIR19B1 , and MIR92A1; Supplementary Data 7 ; Fig. 2 ) [25] . Likewise, four long intergenic non-protein-coding RNAs were affected ( LINC01049 , LINC00410 , LINC00380 , and LINC00379; chr13:90493288-91211698). On chromosome 1, we identified a region that was deleted in 8% of all pediatric patient samples, covering E2F2 and ID3 . In addition, we detected deletions in 10% of the pediatric cohort of BLK (8p23.1) and CLECL1 (12p13.31) that are exclusively expressed in B cells. Fig. 2: Somatic copy number aberrations (SCNAs). Significant recurring SCNAs are displayed as blocks, based on 72 pediatric cases (55 BL and 17 B-AL cases). Curves indicate residual q -values by GISTIC 2.0 after explaining broad aberrations (Supplementary Data 7 ). A Focal deletions affecting E2F2 and ID3 were detected. B The most consistently observed SCNA contains GPC5 ( q = 1.8e-9). Notably, the non-protein-coding MIR17HG cluster directly precedes this gene and is also affected by these gains and amplifications (Supplementary Data 6 ). *: might represent benign (germline) copy number variants. Full size image Recurrent SNV/indels of ID3 are more frequent in the pediatric cohort ID3 was found to be mutated in 76% of all pediatric cases, but only in 40% of adult samples ( P = 2e-9, Supplementary Data 8 , Figs. 1 , 3A ), which implies a more important role for ID3 in the biology of BL/B-AL in children [6] , [26] . Similarly, SNV/indels affecting the ID3-TCF3-CCND3 pathway were more frequent in children than in adults (87% versus 63%, P = 2e-6; Supplementary Fig. 4A, B ). Hotspot SNV/indels of ID3 were similar between pediatric and adult BL/B-AL, mostly located within the HLH domain (aa 42–85) and mainly characterized as missense, nonsense, or frameshift SNV/indels (Supplementary Data 9 and Supplementary Fig. 4C ). The most frequent SNV/indel L64F in ID3, was found in 21% of pediatric samples and in 12% of adult cases, followed by P56S, identified in 10% of pediatric patients and 4% of adults. Both are thought to act as loss-of-function mutants and contribute to an increased expression of TCF3, as well as subsequent CCND3 activation (Supplementary Fig. 4D, E ) [6] , [10] , [26] . CCND3 itself displayed a frameshift mutation hotspot R271Pfs*76 detected in 15% of pediatric and 6% of adult cases. Fig. 3: Age dependency of the mutation profile. A Comparison of mutation counts between age groups, using the usual age cutoff of 18 years for adult patients. Mutations in ID3 , DDX3X , SMARCA4 , GNA13 , ARID1A, and PTEN are significantly more frequent in pediatric patient samples, while BCL2 , YY1AP1 , PIM1 , CREBBP , CARD11 , SOCS1, and DTX1 are significantly more frequently altered in the adult cohort ( P values by one-sided exact Fisher tests, see Supplementary Data 8 for exact P values and FDRs, * P ≤ 0.05, ** P ≤ 0.01, *** P ≤ 0.001). B A cutoff-free enrichment analysis of mutation densities over age largely confirms cutoff-based results but reveals that the main biological transition of the mutational profile occurs later between 25 and 40 years ( P values by one-sided enrichment analysis and permutation test with 1e5 permutations per tail). Full size image BAF (SWI/SNF) complex components ARID1A/SMARCA4 are recurrently mutated in pediatric Burkitt lymphoma The genes encoding ARID1A and SMARCA4 are two components of the BAF complex responsible for gene regulation. They were found to be recurrently mutated in both age groups. However, the mutation rate was significantly higher in the pediatric cohort, with 32% for ARID1A and 35% for SMARCA4 , compared to the adult cohort, with SNV/indels in 19% and 21%, respectively ( P = 0.008 for SMARCA4; P = 0.010 for ARID1A , Fig. 3A ). Overall, SMARCA4 SNV/indels were mostly missense SNV/indels (84/89, 94%) and located in the DEAD-box (aa 750–942, 33%) or helicase (aa 1110–1194, 31%) region responsible for the alteration of chromatin structure in the process of transcriptional regulation. One SMARCA4 hotspot was identified with a mutation frequency of 3% in the pediatric cohort (G1232S, Supplementary Data 9 ). ARID1A showed predominantly nonsense (pediatric: 40%, adult: 42%) and frameshift (40%, 31%) SNV/indels, most of which were unique despite the identification of D1850Gfs*4 and S11Afs*91 in four and two pediatric samples, respectively. Only 3% of pediatric cases showed SNV/indels in both genes, while 64% of the pediatric cohort had a mutation in one of the genes. In the adult cohort, 41% of samples were affected by mutually exclusive SNV/indels of either ARID1A or SMARCA4 ( P = 6e-5 for pediatric versus adult, Supplementary Fig. 5A, B ). DDX3X SNV/indels are predominantly identified in pediatric Burkitt lymphoma Dead box helicase 3 ( DDX3X ) encodes an X-linked RNA helicase found in the nucleus as well as in the cytoplasm and is responsible for transcriptional activation and translation processes [27] . In total, 34% of all pediatric patient samples harbored at least one mutation in this gene compared to 15% in the adult cohort (Fig. 3A , P = 7e-4). Most cases of the complete cohort had a single SNV/indel in DDX3X , six were double mutated and one case had a triple mutation. In total, 13 SNV/indels resulted in truncated proteins, 16 affected splice sites, and 14 introduced frameshift mutations, ultimately resulting in truncated DDX3X with missing functional DEAD-box or helicase domains. Most of the SNV/indels were localized in the helicase domain, which could potentially lead to a loss-of-function phenotype (Supplementary Fig. 6A ). GNA13 SNV/indels are more frequent in pediatric Burkitt lymphoma We found a higher frequency of GNA13 alterations in the pediatric cohort compared to the adult cohort (Fig. 3A , 19% versus 7%, P = 0.0055). Overall, 48% of all SNV/indels in the pediatric cohort were nonsense SNV/indels with truncation mutations early in the N-terminal region of the protein, including eight SNV/indels stopping at Q27/28, which suggests loss-of-function mutations (Q27*: 4%/6% mutation frequency, Supplementary Data 9 , Supplementary Fig. 6B ). Mutual exclusivity of GNA13 and P2RY8 , as reported for DLBCL samples, could not be confirmed in our total cohort as we found SNV/indels in both genes [28] , [29] . While 29% of the pediatric patient samples showed SNV/indels in GNA13 and/or P2RY8 , the adult cohort had a slightly lower mutation rate at 21% ( P = 0.11, cf. Supplementary Fig. 6C, D ). The majority of P2RY8 SNV/indels were located within the transmembrane domain. Loss of function due to misfolded or mislocalized protein appears likely, which has previously been demonstrated for several point mutations (Supplementary Fig. 6E ) [28] . YY1AP1 is predominantly mutated in adult BL Recurrent SNV/indels in YY1AP1 were found in 16% of cases in the adult cohort. The mutation frequency was significantly higher compared to the pediatric cohort (2%, P = 1e-5). YY1AP1 is responsible for transcriptional activation, DNA repair and replication, and is linked to other cancer types [30] . We found three hotspot SNV/indels with mutation frequencies ranging from 8-12% directly adjacent (G23R, V24G, S25A) or in close proximity (S30R, 4%), which were exclusively in the adult cohort (Supplementary Data 9 ). Interestingly, seven of these samples showed a single mutation, while five cases had two or more SNV/indels within these sites. Additional SNV/indels of the S30R site occurred in four cases (Supplementary Data 9 ). A second gene with alterations predominantly occurring in the adult cohort was BCL2 , which was found to be mutated in 11% of the adult BL cohort, while there were no SNV/indels detected in the pediatric cohort (Fig. 3A , P = 4e-6). Furthermore, the adult cohort showed significantly higher mutation frequencies in PIM1 (7%), CREBBP (10%), CARD11 (5%), SOCS1 (6%), and DTX1 (5%, Fig. 3A ). All of these were either undetected or detected at only very low rates in the pediatric cohort. Taken together, our data reveal a distinct difference between the mutational spectrum in pediatric and adult Burkitt lymphoma with respect to specific genes. Cutoff-free mutation density analysis reveals the main transition of the mutational signature occurs between 25 and 40 years In addition to the usual age cutoff for adults at 18 years, we performed a cutoff-free mutation enrichment analysis (Fig. 3B ). Enrichment tests (see “Methods”) confirmed the significance of age biases in genes determined by the Fisher tests above. However, gene mutation densities over age revealed that the biological main transition of the mutational signature surprisingly occurs later, between 25 and 40 years with a median of about 35 years in our study. In particular, ID3 mutation density relative to children falls to about 40% during this transition, and BCL2 mutations did not occur before. In addition, a tendency for lower mutation frequencies in some genes can be seen for children younger than 7 years, including SMARCA4 , FBXO11 , and PCBP1 . In contrast, several other genes including MYC and TP53 did not show any age bias with respect to mutation density. The highest homogeneity of the mutation profile is visible in the age range of about 7–15 years. Associations of distinct SNV/indels with clinical characteristics of Burkitt lymphoma Associations of genetic markers with clinical data of pediatric Burkitt lymphoma are still scarce and are urgently needed to identify ways for therapy improvement. To this end, we systematically tested for such associations (Supplementary Data. 8 ). Only tendencies to slightly higher rates of SNV/indels in TP53 ( P = 0.044) and SMARCA4 ( P = 0.01) were observed in adolescents of 10–18 years compared to younger children (Fig. 4A ). This is consistent with our mutation over age analysis suggesting a homogeneous mutation signature from about 7–15 years of age. Fig. 4: Mutational frequencies associated with clinical characteristics. For the pediatric cohort, gene mutation rates were associated with the following clinical characteristics: age dependency ( A ); sex ( B ); BM (bone marrow, C ); B-AL vs. BL ( D ); and, central nervous system (CNS, E ). F shows the sex-specific differences in the adult cohort. FOXO1 , BCL2 , and CREBBP are predominantly found in the female cohort, while MYC , SMARCA4, and DDX3X are overrepresented in the male cohort ( P values by one-sided exact Fisher tests, see Supplementary Data 8 for all P values and FDRs, * P ≤ 0.05, ** P ≤ 0.01, *** P ≤ 0.001. Full size image Strikingly, DDX3X showed a very strong bias to male patients, of 46%:4% incidence compared to females (Fig. 4B , P = 4e-10). CCND3 SNV/indels were significantly more frequent in cases with bone marrow (BM) involvement or Burkitt leukemia (Fig. 4C , P = 0.003). In contrast, SNV/indels in GNA13 showed an incidence of only 4%:32% in B-AL, i.e., was significantly less frequent (Fig. 4D , P = 6e-7). Likewise, cases with SNV/indels in GNA13 were less likely to have CNS involvement at diagnosis (Fig. 4E , 5%:23%, P = 0.007). As the information on clinical parameters for the adult patients was limited, the analysis was restricted to differentiation by sex. Again, a male predominance for SNV/indels in DDX3X was observed, but only by 3%:22% and with a relatively high false discovery rate due to lower case numbers (Fig. 4F , P = 0.006). TP53 mutation status is associated with inferior outcome in pediatric patients The overall survival for pediatric patients with SNV/indels in TP53 was significantly inferior to patients with TP53 wild-type (Figs. 5 A, 6A ). To exclude effects from other events (e.g., treatment-related deaths, etc.) further analyses focused on the cumulative incidence of relapse. SNV/indels of TP53 were significantly associated with a cumulative incidence of progression or relapse of 25 ± 4%, compared to 6 ± 2% for BL with TP53 wild-type status (Fig. 5B , P = 0.0002). Remarkably, a higher number of TP53 SNV/indels per case was not correlated with a higher cumulative incidence of relapse (Supplementary Fig. 7A ). The pediatric cohort comprised 40 patients, who received rituximab in addition to chemotherapy according to the NHL-BFM treatment protocol. The prognostic relevance of TP53 SNV/indels could also be observed in the rituximab cohort (Supplementary Fig. 7B ). Fig. 5: Mutations associated with survival and cumulative incidence of relapse in the pediatric cohort. A The overall survival for pediatric patients with SNV/indels in TP53 was significantly inferior to patients with TP53 wild-type (Kaplan–Meier survival estimation, log-rank test). B TP53 mut cases also showed an increased risk of relapse (cumulative incidence, Gray’s test [20] , no adjustments for multiple comparisons in this descriptive context). C Mutations in PCBP1 show a tendency toward prognostic relevance. D Cases with lymphomas harboring MYC and PCBP1 mutations are characterized by an increased risk of relapse. Gains or amplifications on 13q31 specific to GPC5/MIR17HG were significantly associated with a higher risk of relapse ( E ). The lowest incidence of relapse (0/38 cases) was observed for the TP53 wt sub-group and mutations in FBXO11/FOXO1 ( F ). Full size image Fig. 6: Mutational overview of TP53 , PCBP1 , FBXO11, and FOXO1 at the amino acid level in the adult (top) and pediatric (bottom) cohort. A TP53 shows an accumulation of known hotspots at R175, R248, R273, R282, and G245 as found in other malignancies. B PCBP1 shows a hotspot truncation mutant (Y183*) identified in both age groups. C FBXO11 alterations are unique except for W112*. Most mutations were found in the β-helix domain. D In total, 7 4% of all pediatric FOXO1 mutations span the Akt phosphorylation motif on R19, R21, and T24. Exon boundaries are indicated using dashed lines. Full size image The mutational status of PCBP1 tended to be associated with an increased incidence of relapse as well (Fig. 5C , 26 ± 8% vs 14 ± 3%, P = 0.08). Interestingly, all patients with PCBP1 mutation who suffered relapse also showed MYC alterations (Fig. 5D , 13 ± 3% vs 31 ± 9%, P = 0.018). As PCBP1 was shown to interact with MYC and regulate its IRES-dependent expression, it is possible that the truncation mutant Y183* of PCBP1 identified in seven out of eight relapse cases might have an impact on MYC expression (Fig. 6B and Supplementary Data 9 ) [31] , [32] . Very interestingly, we discovered with respect to SCNAs that the highly specific focal gains and amplifications of GPC5/MIR17HG were also significantly associated with inferior survival (Fig. 5E , P = 0.024). For cases with available SNP measurement, 6/13 cases showing this GPC5/MIR17HG lesion relapsed, whereas only 10/59 relapsed without (53% versus 83% relapse-free follow-up). Of the 13 cases with GPC5/MIR17HG lesions, 11 also had a TP53 mutation. Of these double-hit cases, 5/11 relapsed (55% relapse-free follow-up). In contrast, of the 29 cases in our study with TP53 mutation but without GPC5/MIR17HG copy gain, only 7 relapsed (75% relapse-free follow-up). While these numbers hint to a double-hit BL subtype with a very high relapse probability, this hypothesis requires further validation with larger case numbers. Notably, we observed a good-risk sub-cohort of 38 samples (20%) without relapses for patients with TP53 wt status and additional FOXO1 and/or FBXO11 mutations ( P = 0.05, Figs. 5 F, 6C, D ). In general, the process of BL lymphomagenesis is thought to depend on three different important pathways that are partially interconnected: escape of apoptosis, deregulated PI3K signaling, and changes in the cell cycle leading to proliferation and survival of cancer cells [33] . In all cases of BL/B-AL pathogenesis, deregulated MYC signaling is a main driver. Due to MYC mutation, proliferation and apoptosis are uncoupled, consequently proliferation is stimulated and apoptosis abrogated. Deregulation and progression of cell cycle is augmented by several mutations, for example by a mutation in CCND3 , TCF3 , ID3 , and TP53 [9] , [26] , [34] , [35] . Here, we analyzed a large cohort of pediatric BL, based on high-quality DNA from fresh-frozen samples and an analysis pipeline validated by comprehensive Sanger sequencing, to have a calling sensitivity of 0.993 and specificity of 0.989. We systematically compared the mutational spectrum with adult BL as only limited information on the differences/similarities to pediatric cohorts are available [22] , [36] . In addition to the well-known MYC driver we identified recurrent SNV/indels in the ID3 - TCF3 - CCND3 pathway in 87% of cases as a potential second hit in our pediatric cohort. This is in contrast to the adult cohort, in which alterations of the ID3 - TCF3 - CCND3 pathway were identified in only 63%. However, SNV/indels of BCL2 or YY1AP1 were nearly exclusively identified in adult BL cases. Our cutoff-free analysis of the mutation landscape over age suggests that the biological transition of mutational profile occurs between 25 and 40 years, i.e., later than the typically assumed adult threshold. The question of why more male patients are affected by BL remains unanswered. Therefore, we analyzed gender-specific alterations in both cohorts and, strikingly, found a very strong bias of DDX3X mutations towards male individuals, which was very recently confirmed by Gong and colleagues [37] . In total, 64% of all SNV/indels identified in the pediatric relapse cohort were nonsense or frameshift variants of DDX3X , thought to decrease the expression level of DDX3X. ARID1A and SMARCA4, two subunits of the SWI/SNF complex, were frequently targeted by mutations in pediatric BL samples. For ARID1A, a functional compensation by ARID1B and ARID2 has recently been shown [38] . Hence, it would be reasonable to analyze these genes or other members of this complex in future studies to determine if they can indeed functionally compensate for the loss of function of ARID1A, as suggested by our mutational analysis. Interestingly, SNV/indels of genes encoding SWI/SNF components result in increased activity of the histone methyltransferase EZH2, which can be targeted by EZH2 inhibitors such as tazemetostat. Tazemetostat shows promising activity in aggressive B-cell lymphoma, such as r/r GCB-type DLBCL, especially when EZH2 is mutated [39] , [40] . In addition, loss of the SWI/SNF subunit ARID1A is further reported to be associated with increased sensitivity to PI3K/Akt inhibition in cancer. However, the role of this potential crosstalk mechanism in lymphoma is as yet unclear [41] , [42] . In DLBCL, SNV/indels of FOXO1 or FBXO11 are linked to a higher relapse rate [43] , [44] . Notably, the pediatric BL sub-group with the most favorable prognosis in this study were patients with SNV/indels in FBXO11 or FOXO1 on a TP53 wt background. The T24I mutation of FOXO1 identified in pediatric patient samples may lead to an escape of the BCR/PI3K signaling phosphorylation site required for nuclear localization and subsequent expression of target genes [45] . As most SNV/indels are in close proximity to this phosphorylation site, they may have similar effects on the phosphorylation state or transcriptional activity of FOXO1 [46] . Taken together, it seems possible that FBXO11, as the direct interaction partner of TP53 responsible for its neddylation and subsequent degradation, and FOXO1 influence survival and proliferation [47] . The least favorable prognosis in this study with a relapse-free follow-up of only 55% was observed for cases double-hit by a TP53 mutation and simultaneous copy gain or amplification of GPC5/MIR17HG . Interestingly, increased expression of MIR17HG has already been assigned to inferior outcome in BL [48] . Mechanistically, MIR17HG overexpression leads to the downregulation of PTEN, ultimately resulting in increased PI3K/Akt signaling [49] , [50] . A key finding of this study is that the prognostic relevance of recurrent SNV/indels affecting TP53 is in line with our previous clonal evolution data, which point to missing TP53 wt protein expression levels in lymphoma samples [11] . The relevance of this finding is underlined by the findings from refs. [35] , [51] , which were published during the revision of this study [36] , [51] . Both studies show the negative impact of TP53 mutations on survival. The results of these independent studies validate each other and pave the way for rapid translation into upcoming clinical trials by targeting malfunctioning TP53 directly. One strategy might be the inhibition of upstream regulators MDM2 and MDM4 , to decrease the ubiquitination and subsequent proteasomal degradation of TP53 wt . In addition, eprenetapopt, which was recently positively evaluated in a study of patients with MDS, could be a promising drug to restore the TP53wt level [52] . However, the impact of these drugs on mutated TP53 in BL must be verified in vitro and in vivo. In summary, restoring the TP53 wt level could also decrease MYC expression and initiation of apoptosis. Taken together, we provide a detailed comparison of BL in different age groups that will contribute to a sub-group-specific understanding of BL biology and future treatment options. Samples and cell lines This study complies with all relevant ethical regulations and was approved by the ethics committee of the medical association Westfalen-Lippe, Germany, and the University of Muenster, Germany (pediatric cohort: 2015-495-f-S, adult cohort: 2017-534-f-S). In total, fresh-frozen samples of 298 mature B-cell lymphoma for 191 pediatric BL patients, 97 adult BL patients, and 10 BL cell lines were evaluated (Supplementary Fig. 8 ). For 86 of the 191 sequenced pediatric BL or Burkitt leukemia (B-AL) cases, additional paired fresh-frozen germline samples were available. All 191 pediatric cases were registered in the NHL-BFM data center and received confirmation of diagnosis by central reference laboratories of the NHL-BFM study group. Pediatric tumor samples were reviewed by expert hematopathologists and classified according to the WHO 2016 guidelines. They were treated according to the consecutive uniform protocols NHL-BFM95, B-NHL BFM04 or NHL-BFM Registry 2012 [53] . Clinical data for pediatric patients were obtained from the NHL-BFM study center in Münster, Germany. Molecular features of 18 of the 191 pediatric cases have been described already in previous publications of the ICGC MMML-Seq consortium [8] , [11] . For the analyses of adult BL, samples were contributed by experienced laboratories for 97 adult BL patients. Written informed consent was obtained from all patients and/or their legal guardians. Patients did not receive any financial compensation for participation. Cell lines Blue-1, Daudi, Dogkit, Gumbus, Jijoye, Raji, and Ramos were obtained from Louis Staudt (National Cancer Institute, Bethesda). Namalwa and BL-60 were obtained from Stephan Mathas (Max Delbrueck Center, Berlin). BL-70 was obtained from the DSMZ, Braunschweig, Germany (catalog number ACC 233). Tissue handling DNA was extracted from fresh-frozen tumor tissue, bone marrow, or effusion samples using the DNeasy Blood and Tissue kit (Qiagen, Hilden, Germany). For the isolation of corresponding germline DNA, peripheral blood or bone marrow without blast infiltration was used. 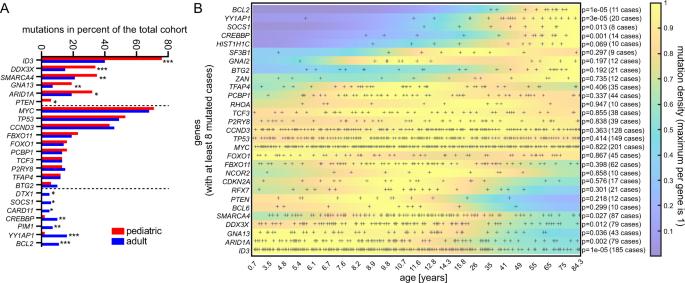Fig. 3: Age dependency of the mutation profile. AComparison of mutation counts between age groups, using the usual age cutoff of 18 years for adult patients. Mutations inID3,DDX3X,SMARCA4,GNA13,ARID1A,andPTENare significantly more frequent in pediatric patient samples, whileBCL2,YY1AP1,PIM1,CREBBP,CARD11,SOCS1,andDTX1are significantly more frequently altered in the adult cohort (Pvalues by one-sided exact Fisher tests, see Supplementary Data8for exactPvalues and FDRs, *P≤ 0.05, **P≤ 0.01, ***P≤ 0.001).BA cutoff-free enrichment analysis of mutation densities over age largely confirms cutoff-based results but reveals that the main biological transition of the mutational profile occurs later between 25 and 40 years (Pvalues by one-sided enrichment analysis and permutation test with 1e5 permutations per tail). Targeted deep sequencing and data analysis Targeted deep sequencing was performed for 134 genes previously identified to be recurrently mutated in BL/B-AL (Supplementary Table 3 ). Previous publications and publicly available data from the International Cancer Genome Consortium ( www.ICGC.org ) were screened for genes with recurring genomic alterations (≥ 2 SNV/indels in the same gene). A Nextera rapid capture custom kit was designed using the Illumina DesignStudio. For every gene, all regions in which previous SNV/indels had been described were covered. For 40 of these genes, the entire coding sequence was covered because previously described alterations were scattered over the entire coding sequence or they were exceptionally frequently affected by SNV/indels according to previous reports. Exact positions of all probes used for enrichment are listed in Supplemental Data 2 . Library preparation was performed according to manufacturer recommendations (Illumina, San Diego, USA). Qubit dsDNA assay and Bioanalyzer High Sensitivity DNA chips were used for DNA quantification and library validation. Targeted deep sequencing was performed on a MiSeq-Sequencer using MiSeq Reagent Kit v2 (300 cycle) with 24 samples per run. An overview of our analysis pipeline with integrated methods and utilized external databases is shown in Supplementary Fig. 1 ; key steps are described next. All somatic mutations are provided in Supplementary Data 2 . Sequence alignment Measured sequence reads were preprocessed and quality-controlled using cutadapt 1.16, Trim Galore! 0.5.0 and FastQC 0.11.5 [54] , [55] , [56] . Trimmed reads were aligned against the current human reference genome from the Genome Reference Consortium (GRCh38) using HISAT2 v2.0.4 [57] , [58] . Variant discovery, quality control on read and sample level, final cohort sizes For variant discovery, we utilized the Genome Analysis Toolkit v4.0.6.0 [59] and Mutect2 [60] . Only reads aligned by HISAT2 that also passed GATK and Mutect quality control filters were utilized for subsequent variant discovery. Basic variant filtering To build a panel of normal variants (PON) [61] , we performed variant discovery with the same experimental and analytical pipeline for all normal controls. A variant was included in the PON if Mutect determined it as significant in at least two independent subjects. This PON was subsequently used to filter germline variants and potential pipeline-specific artefacts when applying Mutect. For tumor samples for which DNA sequencing of paired normal cell samples was available, we additionally utilized matched normals for a more specific paired statistical variant analysis by Mutect. Otherwise, we used the unpaired analysis mode. In addition, we used the gnomAD database as large population germline resource based on the Exome Aggregation Consortium ExAC [62] for basic filtering. Variant annotation and advanced filtering Next, we applied an optimized multistage filter hierarchy to reach maximal specificity of somatic mutation calls. All filter steps in the applied order are listed in Supplementary Data 3 . For this hierarchy, we annotated discovered variants with their transcript and protein level consequences using TransVar 2.4.0 [63] and the NCBI RefSeq gene models [64] . In case of multiple RefSeq transcripts per gene, we annotated each variant with the one leading to the strongest possible biological consequence on protein level according to TransVar. For mutation overview plots, we selected the first principal transcript of the respective gene according to the APPRIS database [65] . In addition, we annotated variants with confirmed somatic mutations according to the Catalogue Of Somatic Mutations In Cancer (COSMIC v85) [61] , the NCBI database of common human variants (>=5%) in any of the five large populations from dbSNP build 151 [66] , and NCBI ClinVar [67] (version 2018-04) using vcfanno v0.3.0 [68] . Variants called somatic Based on variant statistics from Mutect, GATK, and all annotations, our filter hierarchy called 0.25% of all variants in this targeted panel as somatic mutations for the pediatric sub-cohort, i.e., 7.32 on average per sample. For adult BL patients, 0.33% were called somatic (8.49 per sample) whereas for cell lines, 0.52% were called somatic (13.29 per sample). See Supplementary Data 3 for detailed mutation counts and percentages remaining after each filtering step. Identification of cancer genes by mutation abundance To test if genes depicted in our oncoplots (with > =10% cohort mutation frequency, Fig. 1a, b ) were positively selected by mutation processes, we applied the dNdScv tool to all somatic mutations (including synonymous ones) [24] . All oncoplot genes except for TCF3 had a dN/dS ratio significantly greater than 1 (q dNdS < =0.1), suggesting an excess of coding mutations (Supplementary Data 5 ). The likely reason for the negative result for TCF3 is alternative transcripts. We discovered 40 missense mutations for NM_001136139 [ https://www.ncbi.nlm.nih.gov/nuccore/NM_001136139 ] ( TCF3 transcript variant 2, protein variant NP_001129611 [ https://www.ncbi.nlm.nih.gov/protein/NP_001129611 ]), whereas only 2/40 were counted by dNdScv, as 38/40 are intronic in context of the default transcript NM_003200 [ https://www.ncbi.nlm.nih.gov/nuccore/NM_003200 ]. Additional tools and software utilized for sequencing analysis For various analysis tasks in the sequencing pipeline, we used bedtools [69] , the Integrated Genomics Viewer [70] , the Picard toolkit [71] , and SAMtools [72] . For analysis pipeline orchestration including parallel remote analysis jobs on high-performance clusters as well as for most visualizations including oncoplots, we used MATLAB ® (versions R2018a-R2020a, The MathWorks ® Inc., Natick, Massachusetts, USA). R (version 3.6.3, R Foundation for Statistical Computing, Vienna, Austria), Python (version 2.7-3.X, Python Software Foundation, Wilmington, Delaware, USA), and GNU parallel were used for running various tools or for local parallelization [73] . Needle plots of mutation profiles were created using ProteinPaint [74] . 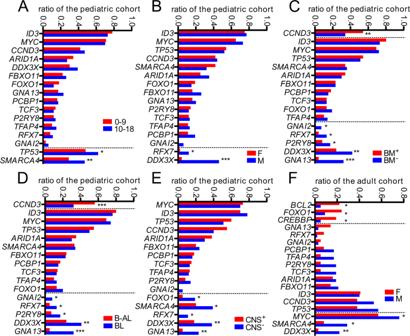Fig. 4: Mutational frequencies associated with clinical characteristics. For the pediatric cohort, gene mutation rates were associated with the following clinical characteristics: age dependency (A); sex (B); BM (bone marrow,C); B-AL vs. BL (D); and, central nervous system (CNS,E).Fshows the sex-specific differences in the adult cohort.FOXO1,BCL2, andCREBBPare predominantly found in the female cohort, whileMYC,SMARCA4,andDDX3Xare overrepresented in the male cohort (Pvalues by one-sided exact Fisher tests, see Supplementary Data8for allPvalues and FDRs, *P≤ 0.05, **P≤ 0.01, ***P≤ 0.001. 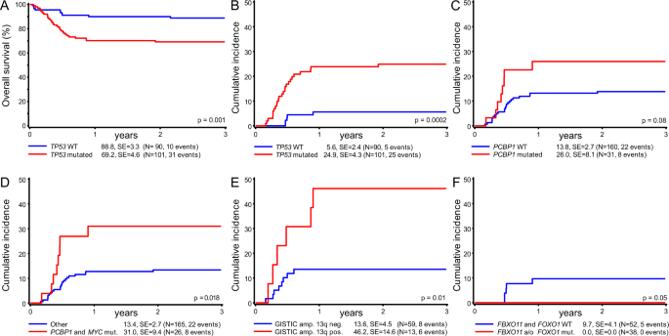Fig. 5: Mutations associated with survival and cumulative incidence of relapse in the pediatric cohort. AThe overall survival for pediatric patients with SNV/indels inTP53was significantly inferior to patients withTP53wild-type (Kaplan–Meier survival estimation, log-rank test).BTP53mutcases also showed an increased risk of relapse (cumulative incidence, Gray’s test20, no adjustments for multiple comparisons in this descriptive context).CMutations inPCBP1show a tendency toward prognostic relevance.DCases with lymphomas harboringMYCandPCBP1mutations are characterized by an increased risk of relapse. Gains or amplifications on 13q31 specific toGPC5/MIR17HGwere significantly associated with a higher risk of relapse (E). The lowest incidence of relapse (0/38 cases) was observed for theTP53wtsub-group and mutations inFBXO11/FOXO1(F). All used tools are summarized in Supplementary Table 4 . Validation by Sanger sequencing Validation by Sanger sequencing was performed for a subset of the 191 pediatric patient samples and cell lines; the genes ID3 , CCND3, and TCF3 were sequenced in 72/191 pediatric patient samples [6] . 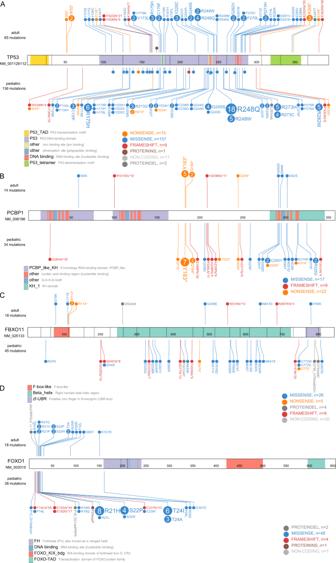Fig. 6: Mutational overview ofTP53,PCBP1,FBXO11,andFOXO1at the amino acid level in the adult (top) and pediatric (bottom) cohort. ATP53shows an accumulation of known hotspots at R175, R248, R273, R282, and G245 as found in other malignancies.BPCBP1shows a hotspot truncation mutant (Y183*) identified in both age groups.CFBXO11alterations are unique except for W112*. Most mutations were found in the β-helix domain.DIn total,74% of all pediatricFOXO1mutations span the Akt phosphorylation motif on R19, R21, and T24. Exon boundaries are indicated using dashed lines. TP53 was sequenced in 57 cases, FOXO1 and FBXO11 in 25, PCBP1 in 13, and P2RY8 in 12/191 cases (for selected primers, see Supplementary Table 6 ). Sequence analysis was conducted by LGC genomics GmbH, Germany. We performed a 1:1 comparison with somatic SNV/indels discovered by targeted DNA sequencing. Before validation, 284 variants were called by Sanger sequencing and/or by the DNA-sequencing pipeline in regions covered by Sanger sequencing. 243/284 were matches (identical genomic HGVS from both pipelines). An additional 10 were matches after manual review (e.g., HGVS annotation ambiguities). In all, 26/284 were discovered by both pipelines, but filtered by the DNA-seq pipeline; after manual review, the DNA-sequencing filtering was confirmed in each case. For completeness, in the same regions covered by Sanger sequencing, additional 272 variants were discovered by DNA sequencing, but not called due to the filter hierarchy. Notably, two variants discovered by Sanger sequencing were not rediscovered by targeted DNA sequencing (hard false negatives before filtering). This corresponds to a false negative rate of 0.007 and a sensitivity of 0.993. One missing aberration was a mutation in the cell line Namalwa at 1:g.23559108_23559207delinsCTTTGATGCAACCATGGGCAAGTCACTTGTCCCTCTCTGGCCTCAGTTTCCCTAAACCGAGTGAGTGGCAATTTTTAAAAACGTCTGCCAACTCCAGGAC, which might be too long for the sequencing technology or Mutect to recognize. The second aberration from an initial tumor sample was a likewise length outlier: 1:g.23559159_23559248delCAGGGGCTGGCTCGGCCAGGACTACCTGCAGGTCGAGAATGTAGTCGATGACGCGCTGTAGGATTTCCACCTGGCTAAGCTGAGTGCCTC. Finally, three of the 284 somatic SNV/indels called by targeted DNA sequencing were not part of the Sanger validation set. This corresponds to a false positive rate of 0.011 and a specificity of 0.989 for DNA sequencing. However, further manual investigation via visualization in IGV showed that all three were present in the raw targeted sequencing data [70] . For a detailed run-down of this validation of our targeted sequencing measurement and analysis pipeline, including detailed filter reasons for each variant if any, see Supplementary Data 4 . Analysis of somatic copy number aberrations (SCNAs) Single-nucleotide polymorphism arrays were measured by LIFE & BRAIN genomics, Germany, using Human OmniExpress v1.3 (Illumina). Sufficient material for SNP arrays was available for 72 pediatric lymphoma samples and 21 matched germline samples. Raw data were preprocessed according to manufacturer instructions (Illumina Genome Studio v2.0.3) [75] . For allele-specific copy number segmentation at the sample level, we utilized ASCAT v2.4.3. ASCAT also estimated sample ploidy and purity (i.e., the cell fraction originating from aberrant tumor cells, as opposed to non-aberrant bystander cells). Recurrent SCNAs at the cohort level were identified and statistically evaluated using GISTIC 2.0 [76] . Mutation clonality by integrative analysis of targeted sequencing and SNP results To identify potential early mutations in the pathogenesis, we estimated mutation clonality. First, we integrated SNP array results (tumor purity, ploidy, and copy numbers) with variant allele frequencies from the targeted sequencing data to estimate the cancer cell fractions (CCF) that harbor-specific mutations. We utilized the formula: [77] 
    f_CCF := f_VAF/f_purity·((1-f_purity)·n_CN,normal+f_purity·n_CN,tumor)
 (1) where \({f}_{{{{{\rm{VAF}}}}}}\) denotes variant allele frequency, \({f}_{{{{{{\rm{purity}}}}}}}\) denotes tumor purity, \({n}_{{{{{{\rm{CN}}}}}},{{{{{\rm{normal}}}}}}}=2\) assuming diploid normal bystander cells, and \({n}_{{{{{{\rm{CN}}}}}},{{{{{\rm{tumor}}}}}}}\) denotes tumor cell copy numbers as estimated by ASCAT. Then, we defined clonal variants using the established threshold of \({f}_{{{{{{\rm{CCF}}}}}}}\ge 0.9\) [78] . Estimated Cancer Cell Fractions can be found together with all called mutations in Supplementary Data 2 (see column group Variant def./call quality/details for tumor). Statistics and reproducibility No statistical method was used to predetermine sample size; all samples of matching diagnosis with enough available sample material were selected for this study. The experiments were not randomized. Several samples were excluded before the final analysis for QC reasons: five samples from the adult cohort due to <10% of the median mapped read count per sample, six samples from the adult cohort due to potentially mismatching disease entity after pathology revision, one pediatric sample due to cell material issues (very low allele frequencies even at SNP loci), three pediatric samples due to potentially wrong channel assignment or mismatching (tumor, normal) pairs, and one pediatric sample due to NHL as second malignancy. The investigators were not blinded to allocation during experiments and outcome assessment. For binary comparisons between sub cohorts, e.g., pediatric versus adult, and if not otherwise specified, P values were calculated with one-tailed Fisher exact tests. A significance threshold of α = 0.05 was used for all Fisher exact tests (bar graphs). Asterisks indicate significance of single tests as follows: * P ≤ 0.05, ** P ≤ 0.01, *** P ≤ 0.001. In particular, we tested for associations in gene mutation status with age, comparing pediatric (≤18 years) versus adult (>18) patients. Likewise, we tested for significant differences between female and male patients within each age group, as well as the following clinically defined sub cohorts within pediatric patients: <10 years of age versus ≥10 years; with CNS involvement versus without; with bone marrow involvement versus without; and B-AL versus BL. For each comparison, we tested all genes with an overall mutation frequency of at least 2%. False discovery rates (FDR) for sub-cohort comparisons were computed using the Benjamini and Hochberg method over the set of tested hypotheses (genes with at least 2% cohort mutation frequency; cf. Supplementary Data 8 ) [79] . For significance, we used the prescribed error threshold of q = 0.1. Survival analysis The probability of EFS and overall survival (OS) was estimated using the Kaplan–Meier method, and compared between subgroups using log-rank tests. EFS was defined as the time from diagnosis to the first event, including relapse, death by any cause, or second malignancy. OS was defined as the time from diagnosis to death by any cause. Cumulative incidence functions for relapse were constructed using the Kalbfleisch and Prentice method and compared with Gray’s test [20] . For survival data, we performed explorative hypothesis generation by testing various combinations of discovered genetic lesions. Here, no adjustments were made for multiple comparisons. Hence, the resulting significant associations are descriptive, but we consider validation tests for them worthwhile in future independent BL cohorts. Death in remission and secondary malignancy were considered as competing events. All cumulative incidence estimates are given together with their corresponding standard error (±SE). Cutoff-free mutations-over-age analysis To analyze the age profile of mutations, we estimated mutation density with the Statistics and Machine Learning Toolbox (Matlab R2020a, ksdensity command). To account for artefacts at interval borders, we used the data reflection method. To assess the statistical significance of mutation enrichment at either old or young ages in a cutoff-free way, we applied one-sided enrichment analysis [80] with 1e5 permutations per tail, separately for each gene by ranking patients by their age and counting mutated cases as signature members. Reporting summary Further information on research design is available in the Nature Research Reporting Summary linked to this article.